On-the-fly decoding luminescence lifetimes in the microsecond region for lanthanide-encoded suspension arrays Significant multiplexing capacity of optical time-domain coding has been recently demonstrated by tuning luminescence lifetimes of the upconversion nanoparticles called ‘ τ -Dots’. It provides a large dynamic range of lifetimes from microseconds to milliseconds, which allows creating large libraries of nanotags/microcarriers. However, a robust approach is required to rapidly and accurately measure the luminescence lifetimes from the relatively slow-decaying signals. Here we show a fast algorithm suitable for the microsecond region with precision closely approaching the theoretical limit and compatible with the rapid scanning cytometry technique. We exploit this approach to further extend optical time-domain multiplexing to the downconversion luminescence, using luminescence microspheres wherein lifetimes are tuned through luminescence resonance energy transfer. We demonstrate real-time discrimination of these microspheres in the rapid scanning cytometry, and apply them to the multiplexed probing of pathogen DNA strands. Our results indicate that tunable luminescence lifetimes have considerable potential in high-throughput analytical sciences. Fluorescence lifetimes are typically less than tens of nanoseconds; however, materials containing trivalent lanthanide ions usually exhibit longer lifetimes from microseconds to even milliseconds [1] , [2] , [3] . Such materials have been used as luminescent probes and they show improved sensitivity over conventional fluorescence-based methods when time-gated detection is used to remove the autofluorescence background [4] , [5] , [6] , [7] , [8] , [9] . Moreover, recently it was demonstrated that their microsecond-region lifetimes can be fine-tuned to create multiplexing optical codes and assigned to single upconversion nanoparticles [10] , [11] . These tunable lifetime values constitute a new temporal dimension of optical codes for data storage, document security and multiplexing assays, which can simultaneously assess a large number of biomolecular species. The next challenge is centred on the decoding issue—how to read and distinguish the slow-decaying lifetimes of each species at high speed. On the other hand, contemporary life sciences demand new high-throughput analytical technologies, capable of simultaneous identification and quantification of large number of biomolecular species. Suspension arrays are emerging as a future leading technology for multiplexed molecular detection [12] , [13] . They are based on ensembles of microspheres that have been specially coded, most frequently by varying combinations of fluorescent dyes. The microspheres are thus endowed with a range of identifiable colour codes individually assigned to a specific analyte [14] , [15] , [16] . The major advantages of suspension arrays include rapid reaction kinetics, the absence of washing steps, higher sample throughput, as well as reproducible manufacture of microsphere families. Moreover, suspension arrays have potential as quantitative assays owing to the uniform surface of microspheres, the simplicity of use and their reduced expense compared with alternatives. The test panels are flexible to design by simply selecting a different combination of microspheres. Towards these desired advances over the planar array biochips, significant efforts have been devoted to create the diverse signatures (barcodes) on microspheres and to expand multiplexing capacities of suspension arrays [17] , [18] , [19] . In general, although fluorescence encoding and decoding appear to be more practical than non-fluorescence schemes in terms of assay design, cost per test, simplicity and throughput, producing a very large number of independent fluorescence codes by varying the intensity ratios of different colours has been restrained in the crowded spectral domain. In the present work, we identify a fast fitting algorithm based on the method of successive integration (MSI) [20] , [21] , and evaluate its practicability in realising the on-the-fly measurement of luminescence lifetimes with sensitivity down to single microspheres. This enables a powerful lifetime-decoding capability for an on-the-fly scanning cytometry [22] , [23] . In our parallel investigation of this work, we adopt the scheme of luminescence resonance energy transfer (LRET) [24] , [25] , [26] , [27] to continuously tune the luminescence lifetimes of downconversion lanthanide complexes within microspheres for encoding. This complementary lifetime coding and decoding by the downconversion lanthanide luminescence within microspheres immediately enables a new library of optical identities for high-content screening of multiple pathogen DNA strands in high speed. Theoretical analysis The techniques for determining fluorescence lifetimes have been previously developed [28] , [29] , [30] , [31] , [32] , and implemented in the fluorescence-lifetime imaging microscopy [33] , [34] , [35] and the phase-sensitive flow cytometry [36] , [37] , [38] . However, developed for the nanosecond region, they are unsuitable for real-time discrimination of luminescence lifetimes, due to the facts associated with the microsecond region that: (i) the computation time of fitting algorithms increases nonlinearly with the data volume; (ii) an improper detection configuration may lead to significant errors in lifetime measurement; and (iii) various noise sources have to be taken into account in such a long timescale. Consider an ensemble of luminescence probes excited by a pulse where, for simplicity, we assume that the luminescence decay profiles are monoexponential. From a statistical point of view, these probes emit individual photons with the total number (as a function of time) distributed according to a nonhomogeneous Poisson process with the exponential function as its intensity parameter (for explanation see Supplementary Notes 1–3 ). The process of lifetime measurement is, in essence, to calculate the lifetime parameter τ in the exponential function from the luminescence decay by using some kind of statistical estimation. Assuming a decay profile is recorded as the counts of luminescence photons individually collected at M temporal intervals (channels) of the same length T , our aim in this section is to determine the optimal M and T . The Cramér–Rao inequality of the estimation theory indicates that the lowest-possible variance of any unbiased estimator (called Cramér–Rao lower bound, CRLB) is given by the inverse of the Fisher information matrix [39] . In the absence of dark noise, the CRLB for lifetime τ can be explicitly derived (see Supplementary Note 4 ). 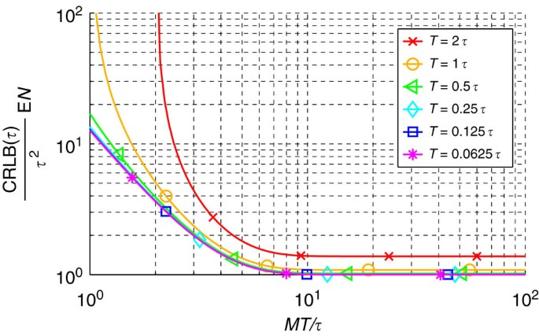Figure 1: Cramér–Rao lower bound for lifetime estimation under different detection channel configurations. CRLB(τ) is normalized by the lifetime (τ2, since CRLB(τ) represents variance) as well as the average number of photons (EN), and plotted as a function ofMT/τ.Tis the width of every detection channel andMis the total number of detection channels, so thatMTindicates the entire length of the detection window. Figure 1 illustrates the relative CRLB normalized by the signal intensity (the expected value of the total number of luminescence photons N ) as a function of MT / τ for different channel widths T . Note that it approaches unity under ideal conditions, which is a feature of the Poisson process. On one hand, since MT is the entire length of the detection window, these curves indicate an essential condition for accurate measurement of lifetime: the detection window should be sufficiently long compared with the lifetime under test. Otherwise, if the window duration is only about the lifetime under test, for example, the variance in the final results will be at least tenfold larger than its actual value, since no algorithm can achieve a lower variance than the CRLB. In practice, eight times the largest-possible lifetime value as the length of detection window is a rule of thumb suggested by Fig. 1 . On the other hand, the decay curves with channel width T smaller than half of the lifetime τ give almost identical results. This indicates that the optimum T for rapid lifetime computation should be around half of the lifetime value under test. Alternatively, if sampling is applied at a high frequency, the lifetime computation can be accelerated simply through a pretreatment of data binning to reduce the channel number, without sacrificing the precision. This is particularly useful when different lifetimes need to be measured and T is set about half of the smallest-possible lifetime value. Figure 1: Cramér–Rao lower bound for lifetime estimation under different detection channel configurations. CRLB( τ ) is normalized by the lifetime ( τ 2 , since CRLB( τ ) represents variance) as well as the average number of photons (E N ), and plotted as a function of MT / τ . T is the width of every detection channel and M is the total number of detection channels, so that MT indicates the entire length of the detection window. Full size image Numerical simulation Having identified the optimum detection configuration for the lowest variance estimation of the decay lifetime, we then compared four leading lifetime fitting algorithms through numerical simulations. The aim of this comparison is to determine which algorithm has the best accuracy and speed. The first method is nonlinear fitting based on maximum-likelihood estimation (MLE-NF), which is reported in the literature as the most accurate algorithm to estimate parameters from exponential decays [40] . The second method (MLE-PR) is a pattern recognition technique comparing Kullback–Leibler minimum discrimination information, which is effectively MLE in the discrete regime [41] , [42] . The third is the rapid lifetime determination (RLD) method, which has been widely applied due to its great simplicity [43] , [44] . The fourth is the MSI, which has attracted recent interest after it was proved to be superior to another popular fast algorithm based on Fourier transform [45] . A detailed description of the numerical simulation can be found in the Methods section, as well as Supplementary Note 5 . 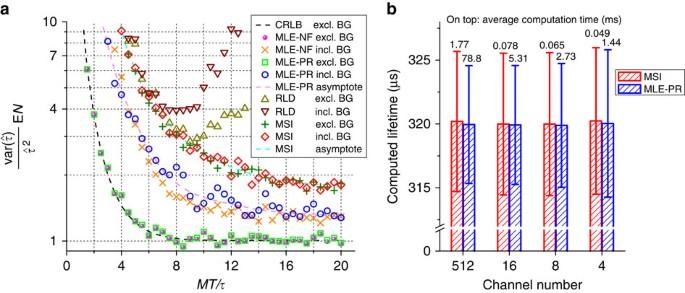Figure 2: Numeric simulation results for lifetime fitting algorithms. (a) The relative variances of lifetime estimators,, normalized by the average number of photons, EN, are shown as a function ofMT/τfor different fitting algorithms with and without background taken into account, alongside the CRLB. (b) Comparison between MSI and MLE-PR methods in terms of accuracy (error bars stand for ±1 s.d.) and computation speed, at different channel numbers as a result of data binning pretreatment. Excl, excluding; incl, including. Figure 2 summarizes the simulation results. Referring to Fig. 2a , when the data curves are free of background noise (consequently no baseline in the exponential function), the variances of the computed lifetimes through both MLE-NF and MLE-PR asymptotically converge to the CRLB—the minimum value they could ever reach statistically. Although not as efficient as MLE, RLD and MSI are similarly good for shorter detection windows; however, with a longer detection window, the MSI obtains better precision while the RLD becomes inefficient. If a background baseline is added to the model (in this case no close form can be derived for the CRLB), MLE-NF is still the most efficient method. The precision of MLE-PR is very close to that of MLE-NF, only slightly inferior. The performance of RLD suggests its inappropriateness for long lifetime measurement, despite the fact that it has been used in a few purpose-built instruments [35] , [46] , [47] . To our surprise, MSI still has the same performance regardless of the background noise. In fact, the difference of precision between MLE-PR and MSI becomes very small as the signal-to-background ratio further decreases (see Supplementary Fig. 1 ). Figure 2b compares the lifetime computation by MLE-PR and MSI with different numbers of channels (true lifetime value τ =320 μs; MT / τ =8). It was obvious that MSI is much faster than MLE-PR in about 46 times under identical conditions, to obtain the same unbiased results with variance only about 1.3 times larger. Figure 2b also verifies that a channel width around half of the lifetime under test (the case of 16 channels here) ensures the best balance between accuracy and speed. Figure 2: Numeric simulation results for lifetime fitting algorithms. ( a ) The relative variances of lifetime estimators, , normalized by the average number of photons, E N , are shown as a function of MT / τ for different fitting algorithms with and without background taken into account, alongside the CRLB. ( b ) Comparison between MSI and MLE-PR methods in terms of accuracy (error bars stand for ±1 s.d.) and computation speed, at different channel numbers as a result of data binning pretreatment. Excl, excluding; incl, including. Full size image On the basis of this analysis, we selected the MSI to determine the microsecond-region lifetimes of individual luminescent targets, which offers almost the highest precision but in a much more rapid fashion than alternative algorithms. In fact, since only requiring about 0.078 ms to calculate each lifetime value, it offers the potential for high-throughput lifetime measurement with >10 4 targets per second. Experimental prototype system The fast lifetime-decoding algorithm based on MSI has been applied to our scanning cytometry. 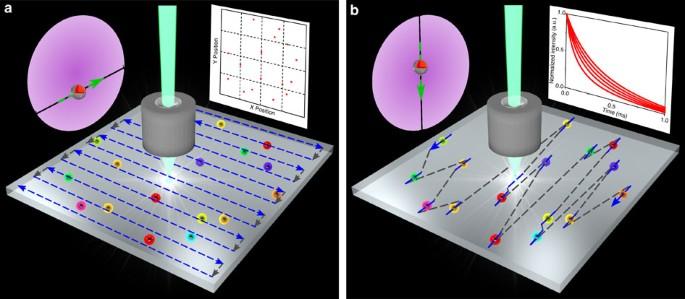Figure 3: Schematics of the time-resolved orthogonal scanning automated microscopy (TR-OSAM). The TR-OSAM can identify micron-sized targets randomly distributed on a microscopic slide, and distinguish them by individuals’ luminescent lifetimes. (a) It typically takes 3 min to scan and map these targets in background-free condition via pulsed excitation and time-gated luminescence detection. The signal trains of luminescence intensity recorded from the detection field-of-view during the transit of the targets are used to obtain their precise locations along the continuous scanning direction. (b) The positional coordinates guide sequential orthogonal scans for spot-by-spot inspection of targets at the centre of the field-of-view, and the luminescence lifetime identity of each target is decoded in real time. Figure 3 shows a schematic diagram of the new time-resolved orthogonal scanning automated microscopy (TR-OSAM) system. The initial scan following the OSAM principle [22] localizes any randomly distributed targets labelled with long-lived luminescence on a slide ( Fig. 3a ). By doing this rapid continuous scan, the wide-field optics can determine the exact positions of each luminescent target. This guides the orthogonal scan along the other direction to be efficient by only following scan lines leading to the preselected targets ( Fig. 3b ), with real-time recording of their luminescence decay profiles during transition. The OSAM operation efficiently extracts the useful data only from target analytes, thus significantly accelerating the process. This further allows real-time computation for lifetimes of individual targets based on their respective waveforms, consisting of luminescence photon counts in M channels of the same length T . The optimized detection configuration of M and T , and the lifetime fitting algorithm implemented in the system, are explained above, while other details can be found in the Methods section. Figure 3: Schematics of the time-resolved orthogonal scanning automated microscopy (TR-OSAM). The TR-OSAM can identify micron-sized targets randomly distributed on a microscopic slide, and distinguish them by individuals’ luminescent lifetimes. ( a ) It typically takes 3 min to scan and map these targets in background-free condition via pulsed excitation and time-gated luminescence detection. The signal trains of luminescence intensity recorded from the detection field-of-view during the transit of the targets are used to obtain their precise locations along the continuous scanning direction. ( b ) The positional coordinates guide sequential orthogonal scans for spot-by-spot inspection of targets at the centre of the field-of-view, and the luminescence lifetime identity of each target is decoded in real time. Full size image LRET suspension arrays Lifetime-tunable luminescent microspheres were produced through the LRET scheme. A trivalent europium complex of thenoyltrifluoroacetonate Eu(TTFA) 3 [48] , [49] and a hexafluorophosphate salt of cationic coumarin [50] were encapsulated into porous polystyrene beads as donor and acceptor dyes, using a simple method of solvent swelling (see Methods section). When in close proximity, a proportion of excited Eu 3+ complexes in the beads non-radiatively transferred energy to the acceptor dyes [51] , [52] , as a result of the spectral overlap between the donor emission and the acceptor excitation (see Supplementary Fig. 2 ). This led to the reduction of the luminescence lifetime of the Eu 3+ complex at the red emission band around 612 nm. By stepwise varying their concentrations, we manipulated the average donor-to-acceptor distance, making it possible to fine-tune the lifetimes of the microspheres in corresponding steps. 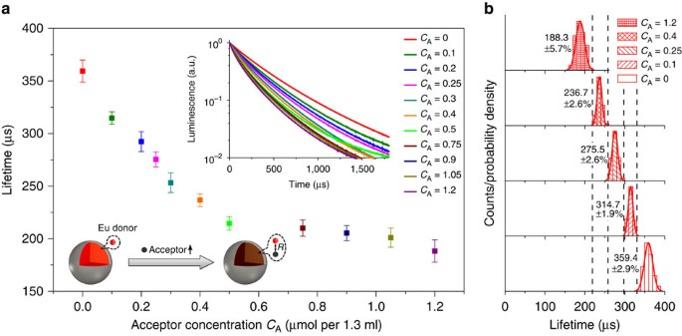Figure 4: Lifetime measurements from individual Eu-containing microspheres engineered by LRET scheme. Different solutions, each having a total volume of 1.3 ml and containing identical amount of Eu complexes (2.5 μmol) as donor but incremental amount of acceptor dyes, were used to produce individual groups of encoded polymer microspheres, followed by TR-OSAM analysis. (a) Luminescence lifetime measured at Eu3+red emission band shortened as the acceptor concentration in the original dye solution increased, as a result of stronger LRET effect. The error bars stand for ±1 s.d. The inset curves are the luminescence decay signals measured from single Eu-LRET microspheres. (b) Among all samples, five types of microspheres gave separate lifetime histograms, so that they can be clearly differentiated in multiplexing assays by the TR-OSAM. The numerals at the left to each histogram are the mean lifetime±the lifetime coefficient of variation for its Gaussian fitting. Figure 4a illustrates that as the acceptor concentration increases (at identical donor concentration), the mean value of donor lifetimes is effectively tuned down from 359 to 188 μs, as measured from individual microspheres by our TR-OSAM. Each lifetime population has a coefficient of variation in the range of 1.9–5.7%. This allows five populations of microspheres to be separated solely based on their lifetimes, with almost no population overlap, as shown in Fig. 4b . Figure 4: Lifetime measurements from individual Eu-containing microspheres engineered by LRET scheme. Different solutions, each having a total volume of 1.3 ml and containing identical amount of Eu complexes (2.5 μmol) as donor but incremental amount of acceptor dyes, were used to produce individual groups of encoded polymer microspheres, followed by TR-OSAM analysis. ( a ) Luminescence lifetime measured at Eu 3+ red emission band shortened as the acceptor concentration in the original dye solution increased, as a result of stronger LRET effect. The error bars stand for ±1 s.d. The inset curves are the luminescence decay signals measured from single Eu-LRET microspheres. ( b ) Among all samples, five types of microspheres gave separate lifetime histograms, so that they can be clearly differentiated in multiplexing assays by the TR-OSAM. The numerals at the left to each histogram are the mean lifetime±the lifetime coefficient of variation for its Gaussian fitting. Full size image These five populations of Eu-LRET microspheres were further mixed together and spiked on a slide area of 15 × 15 mm 2 . After 3 min of scanning by our TR-OSAM, all microspheres were located, with the varying lifetimes of single microspheres computed in real time ( Fig. 5a ). The lifetime histogram ( Fig. 5b ) recovered these five populations with clearly identified boundaries in between, consistent with the results shown in Fig. 4b . Consequently, the TR-OSAM distinguished every type of the Eu-LRET microspheres ( Fig. 5c ). This suggests that these microspheres can create a new type of suspension arrays for multiplexed assays. Through assigning variable lifetime values to the microcarriers, the spectral crosstalk problem can be avoided and the multiplexing levels may be increased further [10] . 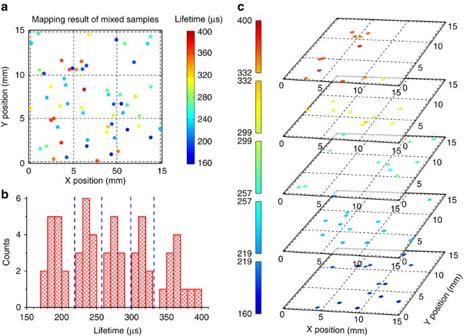Figure 5: Multiplexed detection results of lifetime-encoded microspheres using TR-OSAM decoding. (a) The mapping result of a mixture of five selected types of Eu-LRET microspheres (refer toFig. 4b) showed the locations of individual microspheres on a microscopic slide. Pseudo-colours are used to represent their lifetime values. (b) Each types of microspheres in the mixed sample were recognized based on the separation of lifetime populations using well-defined boundaries in between. (c) The initial mapping result was thus decomposed into five different lifetime ranges for each types of Eu-LRET microspheres carrying lifetime identities. Figure 5: Multiplexed detection results of lifetime-encoded microspheres using TR-OSAM decoding. ( a ) The mapping result of a mixture of five selected types of Eu-LRET microspheres (refer to Fig. 4b ) showed the locations of individual microspheres on a microscopic slide. Pseudo-colours are used to represent their lifetime values. ( b ) Each types of microspheres in the mixed sample were recognized based on the separation of lifetime populations using well-defined boundaries in between. ( c ) The initial mapping result was thus decomposed into five different lifetime ranges for each types of Eu-LRET microspheres carrying lifetime identities. Full size image To further demonstrate the usefulness of this work underpinning the time-domain multiplexing, we carried out a biological experiment for high-throughput simultaneous detection of different pathogen DNAs (single strands). We designed our time-domain suspension arrays (bead assays) to detect four kinds of pathogens—human immunodeficiency virus (HIV), Ebola virus (EV), hepatitis B virus (HBV) and human papillomavirus 16 (HPV-16). The four types of the Eu-LRET microspheres (R-315, R-276, R-237 and R-188; ‘R’ stands for red colour and the numbers refer to the mean lifetime values) were conjugated to the capture probes, respectively, which were the complementary strands for the target DNAs. The other type (R-359) was conjugated to a control DNA probe to verify the specificity of the multiplexed assay. In the detection test, the pathogen DNAs were mixed in one sample and added into the test panel consisting of the five types of conjugated microspheres, followed by adding Qdot 565 as a universal reporter dye (see Fig. 6a for the multiplexing scheme and Methods section for experimental details). The reacted suspension was spread onto a glass slide and analysed by the TR-OSAM. It recovered all the lanthanide-encoded microspheres on the slide by detecting the time-gated luminescence from Eu 3+ complex, and identified their types by decoding the lifetimes in the same colour band ( Fig. 6b ). The reporter fluorescence from Qdot 565 was also measured to confer the presence and amount of the particular target DNAs, indicated by the types of Eu-LRET microspheres ( Fig. 6c ). This result shows that the lifetime-encoded Eu-LRET microspheres can successfully recognize multiple pathogen DNAs in a single test, using the standard format of beads assay. In particular, it is important to note that although the reporter dye is excited by the same light source for the Eu 3+ complex, its fluorescence does not interfere with the encoding luminescence lifetime, due to their complete separation in the temporal domain; while traditional multiplexing techniques based on colour and intensity have to be carefully designed to avoid serious crosstalk issues. 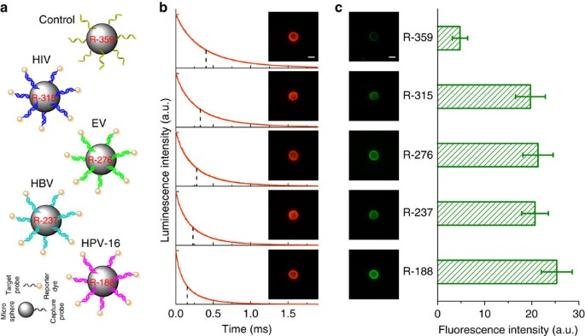Figure 6: Multiplexed DNA detection using lifetime-encoded Eu-LRET microspheres and TR-OSAM decoding. (a) The five selected types of Eu-LRET microspheres (refer toFig. 4b) were conjugated to five different DNA sequences (four of them were complementary to pathogen DNAs from HIV, EV, HBV and HPV-16, and the other was for control purpose). Qdot 565 was used as the universal reporter dye in the beads assay. (b)The microspheres were identified based on their lifetimes measured from Eu3+luminescence decays. (c)The amounts of target pathogen DNAs in the test sample were determined by the reporter fluorescence intensities (error bars stand for ±1 s.d.). Images were taken with different emission filters at 600 ms exposure time under continuous excitation (scale bar, 10 μm). Figure 6: Multiplexed DNA detection using lifetime-encoded Eu-LRET microspheres and TR-OSAM decoding. ( a ) The five selected types of Eu-LRET microspheres (refer to Fig. 4b ) were conjugated to five different DNA sequences (four of them were complementary to pathogen DNAs from HIV, EV, HBV and HPV-16, and the other was for control purpose). Qdot 565 was used as the universal reporter dye in the beads assay. ( b )The microspheres were identified based on their lifetimes measured from Eu 3+ luminescence decays. ( c )The amounts of target pathogen DNAs in the test sample were determined by the reporter fluorescence intensities (error bars stand for ±1 s.d.). Images were taken with different emission filters at 600 ms exposure time under continuous excitation (scale bar, 10 μm). Full size image In principle, the method for lifetime determination presented here is applicable to both the microseconds to millisecond region and the nanosecond region; however, it is in the long lifetime region that this algorithm becomes superior to others for practical circumstances where both high accuracy and high speed are guaranteed. One the other hand, luminescent probes with even longer lifetimes above 1 ms will necessitate extended recording window, thereby less favourable for high-throughput analysis. The microsecond region (that is, 1–1,000 μs) is probably the most advantageous timescale for time-domain multiplexing, since it is sufficiently broad to accommodate a number of lifetime channels while the background interference from autofluorescence and scattering can be completely removed. The feasible time domain also relies on the tunable range of luminescence lifetimes via material engineering, which is currently from tens of microseconds to hundreds of microseconds for both lanthanide-based up- and downconversion probes. It should be noted that the luminescence decays from the LRET microspheres do not exactly follow monoexponential curves, which can be seen from Fig. 4a inset. However, our TR-OSAM based on monoexponential fitting algorithm is sufficient to discriminate different microsphere populations. Also, note that the MSI is applicable to multiexponential cases as well (see Supplementary Note 6 ), which can be integrated for more advanced analytical needs. Moreover, the lifetime codes are independent of either colour in the spectral domain or intensity, and therefore this work also suggests that other LRET microspheres with different emission bands can be simply engineered to further expand the multiplexing capacity of LRET suspension arrays. For example, there are several more spectral bands from the downconversion luminescent or phosphorescent materials [53] , [54] as the potential donors, such as the terbium (Tb) complexes emitting at 490 and 545 nm, dysprosium (Dy) at 580 nm, samarium (Sm) at 600 and 650 nm, and the platinum (Pt) complexes emitting at 700 nm, which can create more lifetime-coding digits through the LRET route. We envisage that this work will lay the foundation to build a library of specific microspheres carrying more than 10,000 codes, to give the users far greater scope and higher flexibility with assay design. Thus, this work unlocks the real potential of suspension arrays as a particularly powerful analytical technique able to cope with the complexity challenges in life sciences and medicine. In summary, we demonstrate both theoretically and experimentally that luminescence lifetimes of microscopic targets in the microsecond region can be measured rapidly and precisely in a simple fashion. This is achieved by the MSI fitting algorithm with an optimized detection configuration. To ensure sufficient accuracy, the key requirements for the detection configuration must be satisfied, that is, the detection window has to be at least eight times of the longest lifetime values under test and the channel width smaller than half of the shortest lifetime under test. Our TR-OSAM system is rapid, sensitive and accurate in resolving the luminescence lifetimes from individual microspheres prepared by the LRET scheme, which can be used to simultaneously probe multiple analytes, such as DNA strands. These results make it possible to take full advantage of the exceptionally long lifetimes offered by luminescent probes, such as lanthanide complexes and upconversion nanocrystals, for multiplexed sensing and imaging in life sciences and photonic applications. Time-resolved orthogonal scanning automated microscopy The TR-OSAM shares the same optical and electronic configurations as the original OSAM reported previously [22] . Briefly, it was modified on an epi-fluorescence inverted microscope (Olympus IX71) to comprise an ultraviolet light-emitting diode (NCCU033A, Nichia; peak wavelength 365 nm, excitation power density ~2.7 W cm −2 in the field-of-view) and a dichroic filter (400DCLP, Chroma) to excite the sample slide placed on a motorized stage (H117, Prior Scientific) through an × 60 objective lens (NT38-340, Edmund Optics). The luminescence signals from the sample were collected by the same objective, split from the excitation optical path by the dichroic mirror, transmit through a band-pass filter (either FF01-607/36 for Eu 3+ luminescence or FF01-560/14 for the reporter fluorescence, both from Semrock) and finally collected by an electronically gateable photon-counting avalanche photodiode (SPCM-AQRH-13-FC, PerkinElmer). The converted electronic photon counts were acquired by a computer at a sampling rate of 500 kHz through a multifunctional data acquisition device (PCI-6251, National Instruments), which also generates synchronised control sequences for time-gated detection as well as stage scanning. On top of the OSAM scheme, the TR-OSAM integrated the lifetime measurement function based on the MSI algorithm and data binning, which were verified by experiments to be appropriate for rapid and robust lifetime computation, especially with data curves superimposed by noise. The period of time-gating cycles was set to 4 ms, consisting of 90 μs excitation pulse, 10 μs time delay and 3,900 μs detection window. The recorded luminescence decay curves were processed by a purposely built LabVIEW program in real time to calculate the lifetimes for individual luminescent targets identified on the slide sample. Numeric simulation to compare lifetime fitting algorithms The mathematic models and computation principles for luminescence lifetime are explained in Supplementary Notes 4 and 5 . The Poisson processes for the time series of a total number 10,000 of the luminescence photon counts were generated from 10,000 random numbers chosen from the exponential distribution with mean parameter of a true lifetime value of 320 μs. The time series were counted within M adjacent channels with all widths equal to T , to obtain a simulated decay curve. A random number chosen from the Poisson distribution with parameter BT ( B =10 5 for Fig. 3 and B =10 6 for Supplementary Fig. 1 ) was superimposed for each channel to simulate the dark counts. For every set of ( M , T ), computation via each fitting algorithm was repeated 1,000 times, each time with a new decay curve. All simulations were executed by a MATLAB program running on a PC with 2.83 GHz quad-core CPU and 4 GB memory. Preparation of Eu-LRET microspheres and slide samples A series of 400 μl dye solutions were prepared, each containing a fixed amount of 2.5 μmol Eu(TTFA) 3 complex (europium tris(thenoyltrifluoroacetonate), 99.9% (rare-earth oxides), Rare Earth Products) and a varied amount of the hexafluorophosphate salt of cationic coumarin ranging from 0 to 1.2 μmol in dichloromethane. Encapsulation of dyes into microspheres was performed through dropwise addition of one dye solution into a 900-μl suspension of polystyrene beads (PC07N/8783, 15.14 μm in diameter, Bangs Laboratories; containing 2.6 × 10 5 beads in ethanol, ultrasonically treated before use). The suspension was stirred for 48 h, and then the dye-containing swollen beads were shrunk in absolute ethanol solvent. After that, the impregnated Eu-LRET microspheres were quickly isolated by centrifugation and washed three times in ethanol:water (vol/vol 1:1), and then stored in 500 μl deionised water. To prepare a test sample for TR-OSAM analysis, a certain amount of suspension typically containing 300~500 Eu-LRET microspheres were drop-cast onto the surface of a glass slide and sealed by a glass coverslip. Multiplexed DNA detection The target DNA sequences of HIV, EV, HBV and HPV-16 were identified from the National Center for Biotechnology Information database. Amino-modified capture DNA oligos and 5′-biotin-conjugated target DNA oligos were purchased from Integrated DNA Technologies (see Supplementary Table 1 for detailed sequences). Each 50 μl of as-prepared Eu-LRET microspheres was used to conjugate each type of capture probes activated by 1-ethyl-3-(3-dimethylaminopropyl)carbodiimide hydrochloride (purchased from Sigma Aldrich) in 2-( N -morpholino)ethanesulphonic acid buffer (50 nM, pH 6.0, purchased from Sigma Aldrich) for 2 h at room temperature. The functionalised microspheres were collected by centrifugation and then mixed to form a test panel. Then, a test sample containing 5 nmol of each pathogen DNA oligos was added into the test panel, and 2 × saline-sodium citrate (purchased from Invitrogen) was used as the hybridization buffer. After 1 h of incubation, the microspheres were washed and resuspended into 100 μl solution containing 10 nM streptavidin-conjugated Qdot 565 (Invitrogen), and then incubated for another 1 h. Finally, the suspension of microspheres was purified and prepared onto a glass slide for analysis by the TR-OSAM. How to cite this article: Lu, Y. et al. On-the-fly decoding luminescence lifetimes in the microsecond region for lanthanide-encoded suspension arrays. Nat. Commun. 5:3741 doi: 10.1038/ncomms4741 (2014).